Graphene-based in-plane micro-supercapacitors with high power and energy densities Micro-supercapacitors are important on-chip micro-power sources for miniaturized electronic devices. Although the performance of micro-supercapacitors has been significantly advanced by fabricating nanostructured materials, developing thin-film manufacture technologies and device architectures, their power or energy densities remain far from those of electrolytic capacitors or lithium thin-film batteries. Here we demonstrate graphene-based in-plane interdigital micro-supercapacitors on arbitrary substrates. The resulting micro-supercapacitors deliver an area capacitance of 80.7 μF cm −2 and a stack capacitance of 17.9 F cm −3 . Further, they show a power density of 495 W cm −3 that is higher than electrolytic capacitors, and an energy density of 2.5 mWh cm −3 that is comparable to lithium thin-film batteries, in association with superior cycling stability. Such microdevices allow for operations at ultrahigh rate up to 1,000 V s −1 , three orders of magnitude higher than that of conventional supercapacitors. Micro-supercapacitors with an in-plane geometry have great promise for numerous miniaturized or flexible electronic applications. Electric double-layer capacitors, also known as supercapacitors or ultracapacitors, store charges only at the electrolyte–electrode interface of active materials through rapid and reversible adsorption/desorption of ions [1] , [2] . Typically, supercapacitors deliver a power density that is an order of magnitude larger (10,000 W kg −1 ) than that of lithium ion batteries, and an energy density that is two orders of magnitude higher (10 Wh kg −1 ) than that of electrolytic capacitors [1] , [2] . Carbon-based materials are currently the most commonly applied electrodes for supercapacitors because they are generally maintenance-free and have an unlimited cycle life [3] , [4] . By far, the most notable progress has been achieved through a deeper understanding of charge storage mechanisms and the development of advanced carbon materials with tailor-made nanostructures [5] , [6] , [7] , [8] . Further improvement of the energy and power densities of supercapacitors, especially at ultrafast rates of <3.6 ms, however, is still a pressing need. Micro-supercapacitors represent one type of the newly developed miniaturized electrochemical energy storage devices. They offer power densities that are several orders of magnitude larger than those of conventional batteries and supercapacitors due to the short ion diffusion length [9] , [10] , [11] , [12] . Importantly, such on-chip microdevices can be directly integrated into other miniaturized electronic devices, such as microbatteries or energy-harvesting microsystems, thereby providing excellent nano-/micro-scale peak power [13] , [14] , [15] . Recently, great efforts have been made to increase the energy and power densities of micro-supercapacitors via the fabrication of nanostructured electroactive materials (such as carbide-derived carbon [10] and carbon onions [11] ), the development of thin-film manufacture technologies (such as electrochemical polymerization [9] , inject printing [16] , and layer-by-layer assembly [17] ) and new device architectures [12] , [18] , [19] , [20] . Nevertheless, micro-supercapacitors that integrate the advantages of the ultrahigh power density of an electrolytic capacitor (10 2 –10 3 W cm −3 ) and the high-energy delivery of a thin-film battery (10 −3 –10 −2 Wh cm −3 ) have not yet been achieved. To this end, it is essential to fabricate thin-film electrodes with a highly accessible electrochemically activated surface area, high electrical conductivity, superior interfacial integrity of the main components (electrode, separator, electrolyte and substrate) and an elaborate device structure with short ion diffusion pathways. Graphene is a robust and attractive electrode material for supercapacitors because of its excellent electrical conductivity, high surface-to-volume ratio, and outstanding intrinsic double-layer capacitance (21 μF cm −2 ) or theoretical capacitance (550 F g −1 ) [21] , [22] , [23] , [24] , [25] , [26] , [27] . Conventional supercapacitors based on curved graphene [24] , activated graphene [25] and laser-scribed graphene [26] as bulk electrodes have been fabricated with greatly enhanced energy densities compared with other carbonaceous materials. Despite much effort towards this aim, the overall performance of graphene-based supercapacitors, especially the power delivery, has not been remarkably improved. Herein we developed a novel class of all solid-state graphene-based in-plane interdigital micro-supercapacitors on both rigid and flexible substrates through micropatterning of graphene films with a nanoscale thickness of 6–100 nm. Due to the high electrical conductivity (345 S cm −1 ) of the fabricated graphene films and the in-plane geometry of the microdevices, the resulting all solid-state micro-supercapacitors deliver a maximum area capacitance of 80.7 μF cm −2 (322.8 μF cm −2 in electrode) and a stack capacitance of 17.9 F cm −3 (71.6 F cm −3 in electrode). Further, they show a power density of 495 W cm −3 , which is the highest value to date for reported supercapacitors, and an energy density of 2.5 mWh cm −3 , which is comparable to that of lithium thin-film batteries, in association with superior cycling stability (≥98.3% capacitance retention after 100,000 cycles). Such in-plane microdevices allow for operations at an ultrahigh scan rate up to 1,000 V s −1 , three orders of magnitude higher than conventional supercapacitors. 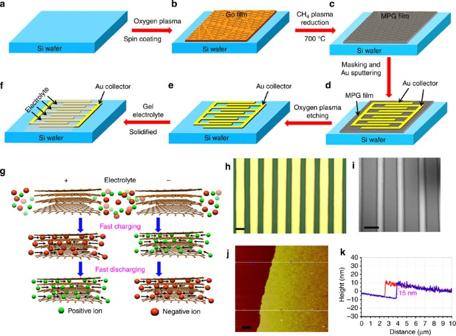Figure 1: Design of MPG-MSCs on a silicon wafer. (a–f) Schematic illustration of the fabrication of MPG-MSCs made up of 30 interdigital fingers integrated onto a silicon wafer. The fabrication process flow includes (a) oxygen plasma surface treatment of silicon, spin-coating of the GO solution on surface-modified silicon, (b) CH4plasma reduction, (c) masking pattern and deposition of gold current collector, (d) oxidative etching in oxygen plasma, (e) drop casting of the H2SO4/PVA gel electrolyte and (f) solidification of the gel electrolyte. (g) In-plane geometry of MPG-MSCs, revealing that the ions between the electrode gaps can be rapidly transported along the planar graphene sheets with a short diffusion length. (h) Optical and (i) SEM images of the microelectrode patterns. Scale bars, 200 μm. (j) Atomic force microscopy image of the MPG film electrode after etching by oxygen plasma and removal of Au by a KI/I2aqueous solution. Scale bar, 1 μm. (k) Uniform thickness of ~15 nm, indicated by the height profile of the MPG film. Fabrication of graphene-based micro-supercapacitors Figure 1 illustrates the fabrication process of the micro-supercapacitors on a silicon wafer. First, a thin film of graphene oxide (GO) ( Supplementary Fig. S1 ) was obtained by spin-coating a GO dispersion (2 mg ml −1 ) on a modified silicon wafer that was first treated with oxygen plasma ( Fig. 1a,b ). Next, the GO film was rapidly reduced by methane (CH 4 )–plasma treatment at 700 °C over a short time (20 s), as indicated by the colour change of the film from yellow to grey ( Fig. 1c ). Structural analysis based on Raman spectra, X-ray diffraction patterns and X-ray photoelectron spectroscopy ( Supplementary Figs. S2–S4 ) revealed the efficient formation of a reduced graphene film (called an MPG film) with a d-spacing of 3.36 Å and a C/O ratio of 9.2. Scanning electron microscopy (SEM) showed that GO films composed of individually stacked sheets were readily transformed into large-area-connected graphene films with a thickness of 15 nm ( Supplementary Fig. S5 ). The resulting MPG films exhibited high electrical conductivity (345 S cm −1 , Supplementary Fig. S6 ), in contrast to 62 S cm −1 for graphene (TG) film thermally reduced at 700 °C for 20 s (see Methods). Subsequently, well-established lithography techniques were applied to manufacture graphene-based interdigital microelectrode patterns through the deposition of gold current collectors, followed by oxidative etching in an oxygen plasma ( Fig. 1d,e ). Optical ( Fig. 1h ) and SEM ( Fig. 1i ) images of the patterned films showed regular widths of 210 μm and an interspace of 70 μm between neighbouring electrode fingers. Atomic force microscopy ( Fig. 1j,k , Supplementary Fig. S7 ) further disclosed the uniform thickness and edge shape of MPG interdigital electrodes. A 5-μl polymer gel electrolyte, such as H 2 SO 4 /polyvinyl alcohol (H 2 SO 4 /PVA), was then drop-casted onto the interdigital electrodes and solidified overnight ( Fig. 1f ). Notably, the gel electrolyte used here not only avoided the harmful leakage of liquid electrolytes, but also reduced the microdevice thickness without additional packaging materials and thus simplified the entire fabrication process. Finally, all solid-state MPG-based micro-supercapacitors (MPG-MSCs) with an in-plane geometry ( Fig. 1g ) were obtained. Figure 1: Design of MPG-MSCs on a silicon wafer. ( a – f ) Schematic illustration of the fabrication of MPG-MSCs made up of 30 interdigital fingers integrated onto a silicon wafer. The fabrication process flow includes ( a ) oxygen plasma surface treatment of silicon, spin-coating of the GO solution on surface-modified silicon, ( b ) CH 4 plasma reduction, ( c ) masking pattern and deposition of gold current collector, ( d ) oxidative etching in oxygen plasma, ( e ) drop casting of the H 2 SO 4 /PVA gel electrolyte and ( f ) solidification of the gel electrolyte. ( g ) In-plane geometry of MPG-MSCs, revealing that the ions between the electrode gaps can be rapidly transported along the planar graphene sheets with a short diffusion length. ( h ) Optical and ( i ) SEM images of the microelectrode patterns. Scale bars, 200 μm. ( j ) Atomic force microscopy image of the MPG film electrode after etching by oxygen plasma and removal of Au by a KI/I 2 aqueous solution. Scale bar, 1 μm. ( k ) Uniform thickness of ~15 nm, indicated by the height profile of the MPG film. Full size image Electrochemical characterization To evaluate the power capability of MPG-MSCs, cyclic voltammetry (CV) experiments were performed at scan rates ranging from 0.01 to 1,000 V s −1 ( Fig. 2 ). Compared with GO film-based micro-supercapacitors ( Supplementary Fig. S8,S9 ), MPG-MSCs exhibited an exceptionally enhanced electrochemical performance with a nearly rectangular CV shape, even at a high scan rate of 100 V s −1 ( Fig. 2a–c ), indicative of the typical double-layer capacitive behaviour. A linear dependence of the discharge current on the scan rate was recognized at least up to 200 V s −1 ( Fig. 2f ). Remarkably, MPG-MSCs charged and discharged rapidly up to 1,000 V s −1 while maintaining excellent capacitance ( Fig. 2a–e ), characteristic of a high instantaneous power. Such rate performance is three orders of magnitude higher than that of electric double-layer capacitors and comparable to any high-power microdevices previously reported [11] . Note that when the thickness of the MPG film is decreased to ~2–3 nm, the scan rate of the microdevice increases, exhibiting a faster response ( Supplementary Fig. S10 ). The cycling performance of MPG-MSCs was examined up to 100,000 cycles at a scan rate of 50 V s −1 ( Supplementary Fig. S11 ). The CV shapes remained almost unchanged and 98.3% capacitance was retained, suggesting extremely stable capacitive behaviour. In addition, MPG-MSCs show the selfdischarge time of 3.3 h from 1.0 to 0.5 V, indicating that the stored charges can be kept for a significant time in such devices ( Supplementary Fig. S12 , Supplementary Note 1 ). 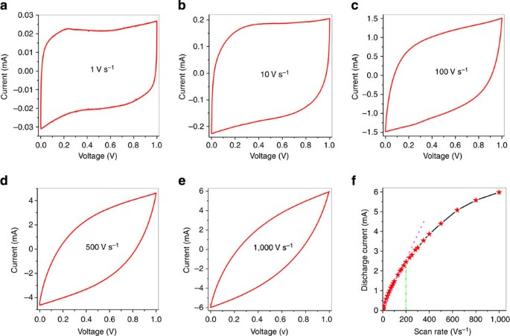Figure 2: Electrochemical characterization of MPG-MSCs on silicon wafer. (a–e) CV curves obtained at different scan rates from 1 to 1,000 V s−1in a H2SO4/PVA gel electrolyte on interdigital micro-supercapacitors with a 15-nm-thick MPG film, showing a typical electric double-layer capacitive behaviour even at different scan rates. (f) A plot of the discharge current as a function of the scan rate (red star line). Linear dependence (magenta dot line) is observed up to at least 200 V s−1(green dash dot line), suggesting the ultrahigh power ability of MPG-MSCs. Figure 2: Electrochemical characterization of MPG-MSCs on silicon wafer. ( a – e ) CV curves obtained at different scan rates from 1 to 1,000 V s −1 in a H 2 SO 4 /PVA gel electrolyte on interdigital micro-supercapacitors with a 15-nm-thick MPG film, showing a typical electric double-layer capacitive behaviour even at different scan rates. ( f ) A plot of the discharge current as a function of the scan rate (red star line). Linear dependence (magenta dot line) is observed up to at least 200 V s −1 (green dash dot line), suggesting the ultrahigh power ability of MPG-MSCs. Full size image To further investigate the superiority of the in-plane device geometry for the performance of MPG-MSCs, we fabricated classical sandwich-supercapacitors comprising H 2 SO 4 /PVA gel electrolytes between two MPG film electrodes (MPG-SSCs, Supplementary Fig. S13,S14 ) with the same MPG film thickness. The area capacitance and stack capacitance of the in-plane MPG-MSCs were calculated to be 80.7 μF cm −2 (322.8 μF cm −2 in electrode) and 17.9 F cm −3 (71.6 F cm −3 in electrode), respectively, both of which were much higher than those of MPG-SSCs (64 μF cm −2 and 1.1 F cm −3 ; Fig. 3a,b ). In addition, MPG-MSCs exhibited a rate capability superior to that of MPG-SSCs. On increasing the scan rates, the capacitances of the MPG-MSCs dropped very slowly. For example, 13.5 μF cm −2 and 3.0 F cm −3 for area capacitance and stack capacitance, respectively, were obtained at 200 V s −1 . Even at an ultrafast rate of 1,000 V s −1 , MPG-MSCs still delivered an area capacitance of 4.5 μF cm −2 and a stack capacitance of 1.0 F cm −3 . In marked contrast, MPG-SSCs gave an area capacitance of only 0.9 μF cm −2 and a stack capacitance of 0.02 F cm −3 at 200 V s −1 . Clearly, the much longer ion diffusion length of MPG-SSCs than that of MPG-MSCs (<180 μm) should be responsible for the lower capacitance at ultrahigh rates ( Fig. 1g , Supplementary Fig. S13 ). To probe the influence of the electrical conductivity of the graphene film on the electrochemical performance of MPG-MSCs, we also fabricated in-plane micro-supercapacitors based on TG film (TG-MSCs, Supplementary Fig. S15,S16 ) without methane–plasma treatment, while keeping the film thickness and cell assembly the same as for MPG-MSCs. The maximum area and stack capacitances (32.6 μF cm −2 and 7.3 F cm −3 ) and rate capability (4.9 μF cm −2 and 1.1 F cm −3 at 400 V s −1 ) obtained for TG-MSCs were much lower than those of MPG-MSCs, indicating that the conductivity of graphene also has an important role in the electrochemical performance. 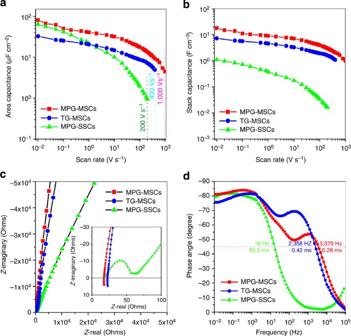Figure 3: Comparison of MPG-MSCs with TG-MSCs and MPG-SSCs. (a,b) Evolution of the (a) area capacitance and (b) stack capacitance versus scan rate. The MPG-MSCs can operate at a higher scan rate of 1,000 V s−1and provide a capacitance 10 times larger than that of the sandwich device, for example, at 200 V s−1, indicating the potential for ultrahigh power delivery. (c) Complex plane plot of the impedance of the microdevices and sandwich device. Inset is a magnified plot of the high-frequency region, showing a vertical intersection with the real axis in MPG-MSCs. (d) Impedance phase angle as a function of frequency for graphene-based microdevices and sandwich device. The −45° phase angle was present at 3,579 Hz for MPG-MSCs, at 2,358 Hz for TG-MSCs and at 16 Hz for MPG-SSCs, demonstrating the fast accessibility of the ions in MPG-MSCs. Figure 3: Comparison of MPG-MSCs with TG-MSCs and MPG-SSCs. ( a , b ) Evolution of the ( a ) area capacitance and ( b ) stack capacitance versus scan rate. The MPG-MSCs can operate at a higher scan rate of 1,000 V s −1 and provide a capacitance 10 times larger than that of the sandwich device, for example, at 200 V s −1 , indicating the potential for ultrahigh power delivery. ( c ) Complex plane plot of the impedance of the microdevices and sandwich device. Inset is a magnified plot of the high-frequency region, showing a vertical intersection with the real axis in MPG-MSCs. ( d ) Impedance phase angle as a function of frequency for graphene-based microdevices and sandwich device. The −45° phase angle was present at 3,579 Hz for MPG-MSCs, at 2,358 Hz for TG-MSCs and at 16 Hz for MPG-SSCs, demonstrating the fast accessibility of the ions in MPG-MSCs. Full size image Electrochemical impedance spectra (EIS) of the micro- and sandwich- supercapacitors are compared in Fig. 3c,3d . Complex plane plots of MPG-MSCs ( Fig. 3c ) exhibit a closed 90° slope at a high frequency, which is characteristic of a pronounced capacitive behaviour. Both MPG-MSCs and TG-MSCs showed a near-vertical line intersection with the real axis at low frequency (inset in Fig. 3c ), indicative of fast ion diffusion in such in-plane microdevices. In contrast, MPG-SSCs featured a high-frequency semicircle with a high charge resistance (41 Ω), attributable to the long ion diffusion pathway for the sandwich device geometry. On the basis of the EIS analysis (inset in Fig. 3c ), MPG-MSCs showed an equivalent series resistance of 17.6 Ω, much lower than that of 22.5 Ω for TG-MSCs. The dependence of the phase angle on the frequency for MPG-MSCs, TG-MSCs and MPG-SSCs is presented in Fig. 3d . The characteristic frequency f 0 at the phase angle of −45° was 3,579 Hz for MPG-MSCs, much higher than that for TG-MSCs (2,358 Hz) and MPG-SSCs (16 Hz). Therefore, the corresponding time constant τ 0 ( τ 0 =1/ f 0 ), which is the minimum time needed to discharge all the energy from the device with an efficiency of more than 50% [11] , [26] , was only 0.28 ms for MPG-MSC, in contrast to 0.42 ms for TG-MSC and 62.5 ms for MPG-SSC. This finding strongly suggests that MPG-MSCs possess enormous potential for the instantaneous delivery of ultrahigh power and energy. Flexible MPG-MSCs We further adapted our fabrication method to construct flexible micro-supercapacitors on a polyethylene terephthalate (PET) substrate. 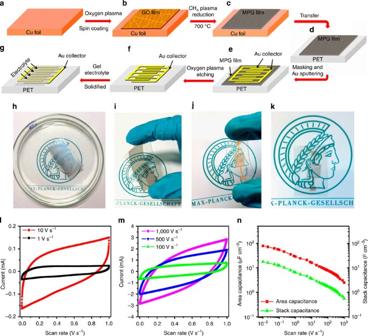Figure 4: Fabrication and characterization of MPG-MSCs-PET. (a–g) Schematic illustration of the fabrication of flexible MPG-MSCs-PET. The fabrication process includes a sequence of (a) spin-coating of GO solution on Cu foil, (b) CH4plasma reduction, (c) transfer of MPG film from the Cu foil to PET substrate, (d) masking pattern and deposition of gold current collector, (e) oxidative etching, (f) drop casting of H2SO4/PVA gel electrolyte and (g) solidification of gel electrolyte. (h–k) Optical images of (h) a 15-nm-thick MPG film (2 × 3 cm) on a polymethyl methacrylate (PMMA) support floated on the water surface after etching Cu foil by aqueous Fe(NO3)3solution, (i) the MPG film transferred onto the PET substrate, (j,k) the resulting MPG-MSCs-PET (j) with and (k) without Au collectors, showing the flexible and transparent characteristics of the fabricated microdevices. (l,m) CV curves of the MPG-MSCs-PET obtained at different scan rates from (l) 1, 10 V and (m) 100, 500 and 1,000 V s−1with a typical electric double-layer capacitive behaviour, even at ultrahigh scan rates, demonstrating its ultrahigh power ability. (n) Area capacitance and stack capacitance of the MPG-MSCs-PET. Figure 4a–g illustrates the fabrication process of MPG-MSCs on a PET substrate (MPG-MSCs-PET). We first produced the MPG film from the spin-coated GO film on Cu foil, followed by CH 4 plasma treatment at 700 °C for 20 s ( Fig. 4a–c ). Subsequently, the MPG film supported by PMMA film was transferred onto the PET substrate (PMMA/MPG/PET) via etching of Cu foil in aqueous Fe(NO 3 ) 3 solution. The PMMA film was removed by acetone ( Fig. 4c,d ). Other fabrication steps, including masking pattern, oxygen plasma etching and addition/solidification of gel electrolyte ( Fig. 4e–g ), were the same as for MPG-MSCs on a silicon wafer (see details in Methods). The optical image of a typical PMMA-supported MPG film (15 nm thick) floated on the water surface is shown in Fig. 4h . An MPG film on the bent PET substrate ( Fig. 4i ) positioned above a logo of the ‘Max-Planck Gesellschaft’ shows the features of large-area uniformity, good transparency and mechanical flexibility. The resulting MPG film had an electrical conductivity of 297 S cm −1 . Importantly, the microdevices can be readily produced with ( Fig. 4j ) and without Au collectors (removed by rinsing in KI/I 2 solution, Fig. 4k ). Figure 4: Fabrication and characterization of MPG-MSCs-PET. ( a–g ) Schematic illustration of the fabrication of flexible MPG-MSCs-PET. The fabrication process includes a sequence of ( a ) spin-coating of GO solution on Cu foil, ( b ) CH 4 plasma reduction, ( c ) transfer of MPG film from the Cu foil to PET substrate, ( d ) masking pattern and deposition of gold current collector, ( e ) oxidative etching, ( f ) drop casting of H 2 SO 4 /PVA gel electrolyte and ( g ) solidification of gel electrolyte. ( h – k ) Optical images of ( h ) a 15-nm-thick MPG film (2 × 3 cm) on a polymethyl methacrylate (PMMA) support floated on the water surface after etching Cu foil by aqueous Fe(NO 3 ) 3 solution, ( i ) the MPG film transferred onto the PET substrate, ( j , k ) the resulting MPG-MSCs-PET ( j ) with and ( k ) without Au collectors, showing the flexible and transparent characteristics of the fabricated microdevices. ( l , m ) CV curves of the MPG-MSCs-PET obtained at different scan rates from ( l ) 1, 10 V and ( m ) 100, 500 and 1,000 V s −1 with a typical electric double-layer capacitive behaviour, even at ultrahigh scan rates, demonstrating its ultrahigh power ability. ( n ) Area capacitance and stack capacitance of the MPG-MSCs-PET. Full size image The electrochemical performance of MPG-MSCs-PET was first examined by CV measurement. Similar to MPG-MSCs, MPG-MSCs-PET can be also operated at an ultrahigh rate up to 1,000 V s −1 ( Fig. 4i,m ). Furthermore, an area capacitance of 78.9 μF cm −2 and a stack capacitance of 17.5 F cm −3 were obtained for MPG-MSCs-PET at 10 mV s −1 , comparable to the performance of MPG-MSCs on a silicon wafer. In addition, the flexible microdevices exhibited excellent cycling stability and mechanical stability. For example, up to 99.1% of capacitance was maintained after 100,000 times at a scan rate of 200 V s −1 ( Supplementary Fig. S17 ), and no capacity degradation was observed when the devices were bent for 100 times. Ragone plot To demonstrate the overall performance of MPG-MSCs, a Ragone plot is shown in Fig. 5 . The data from MPG-SSCs and TG-MSCs, as well as a commercial high-energy lithium thin-film battery (4 V/500 μAh) [11] , high-power aluminium electrolytic capacitor (3 V/300 μF) [26] and Panasonic Li-ion battery (780 mAh, 17 500) [27] are included for comparison. Remarkably, MPG-MSCs delivered a volumetric energy density of 2.5 mWh cm −3 , which is an order of magnitude higher than that of the typical supercapacitors of activated carbon (<1 mWh cm −3 ), and well comparable to that of lithium thin-film batteries (10 −3 –10 −2 Wh cm −3 ) [11] . In addition, MPG-MSCs manifest an ultrahigh power density of 495 W cm −3 (even at a high energy density of 0.14 mWh cm −3 ) discharged within an extremely short time (1 ms). The powder density is at least 50 times higher than that of conventional supercapacitors ( Fig. 5 ), two times higher than that of the state-of-the-art micro-supercapacitors ( Supplementary Table S1 ) and comparable to that of high-power electrolytic capacitors (10 1 –10 3 W cm −3 ) [26] . To the best of our knowledge, this is the first report of micro-supercapacitors with such excellent performance in terms of ultrahigh power and energy densities. 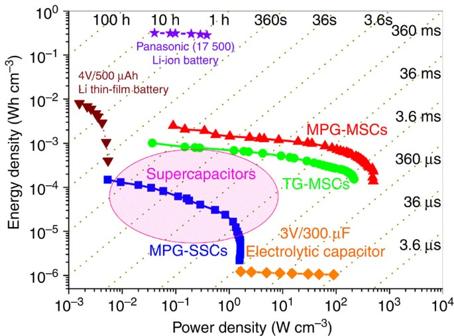Figure 5: Ragone plot of MPG-MSCs. The comparison of energy and power density of MPG-MSCs with TG-MSCs, MPG-SSCs, commercially applied electrolytic capacitors26, lithium thin-film batteries11, Panasonic Li-ion battery27and conventional supercapacitors (indicated by the pink region), demonstrating that MPG-MSCs exhibit exceptional electrochemical energy storage with simultaneous ultrahigh energy density and power density. Figure 5: Ragone plot of MPG-MSCs. The comparison of energy and power density of MPG-MSCs with TG-MSCs, MPG-SSCs, commercially applied electrolytic capacitors [26] , lithium thin-film batteries [11] , Panasonic Li-ion battery [27] and conventional supercapacitors (indicated by the pink region), demonstrating that MPG-MSCs exhibit exceptional electrochemical energy storage with simultaneous ultrahigh energy density and power density. Full size image The superior performance of graphene-based thin-film micro-supercapacitors can be explained by the cooperative effects of the high conductivity of graphene materials and the in-plane geometry of the devices. First, interdigital microelectrodes in MPG-MSCs can maximize the use of the accessible surface area of graphene, which is responsible for the high-charge storage capacity. Second, the MPG film possesses high electrical conductivity ( Supplementary Fig. S6 ), which is another important factor for facilitating electron transport and thus generating high-power supercapacitors. This is because CH 4 plasma reduction can provide an additional carbon source (like C + and CH n + , and CH n , n =1–3) to repair the defects of GO, and therefore give rise to high C/O ratio (9.2) and electrical conductivity (345 S cm −1 ) for MPG film. Last but not least, the in-plane interdigital electrodes in the microdevices allow for ultrafast uptake of the flow of electrolyte ions into or removal from the graphene layers in a short diffusion pathway ( Fig. 1 ) [12] , [28] . Here we demonstrated a prototype ultrahigh-performance graphene-based in-plane micro-supercapacitors. The devices were fabricated based on micropatterning of reduced GO films on both rigid and flexible substrates. The fabrication process is simple, reliable and can be scaled up to pattern hundreds to thousands of devices on one substrate in a relatively short period of time. Such microdevices show ultrahigh volumetric energy densities and power densities operable at ultrafast charge and discharge rates. Improvement of graphene film electrodes, such as film continuity and conductivity ( Supplementary Fig. S18 ), development of new film manufacturing processes, optimization of device configuration (such as increasing interdigital fingers and decreasing the interspaces between the electrodes) and rational selection of electrolytes ( Supplementary Fig. S19 ) will further enhance the performance of the miniaturized micro-supercapacitors. Indeed, MPG-MSCs can also work collaboratively when connected in parallel or in series ( Supplementary Fig. S20,S21 ). Therefore, these miniaturized micro-supercapacitors can offer a nano-/micro-scale power source sufficient to meet certain applications that require higher operating currents and voltages in a short time-frame. Fabrication of an MPG film and device First, GO was prepared from natural graphite by Hummers method as reported in our previous work [29] . Next, GO dispersion (2.0 mg ml −1 ) was sonicated for 2 h and then spin-coated (2,000 r.p.m., 60 s; Headway Research Inc.) on the oxygen plasma-treated silicon wafer (single side polished, 300 nm SiO 2 layer, Si-Mat) using 300 W rf power for 10 min (Plasma System 200-G, Technics Plamsa GmbH), and if necessary the spin-coating steps were repeated to fabricate thick GO film until a desirable film thickness was achieved. The produced GO films were then reduced at 700 °C for 20 s with the methane (CH 4 )–plasma (AIXTRON, Nanoinstruments Black Magic) with a heating rate of 50 °C min −1 . The flow rate of CH 4 gas into the plasma chamber was 100 sccm. The plasma was operated with a 15-kHz waveform drive and ignited with a high-voltage of 800 V. The chamber pressure during plasma treatment was 6.20 Torr. Subsequently, 30 nm of gold (Premion, 99.9985% metals basis, Alfa Aesar) was thermally evaporated (EDWARDS FL400) onto the MPG film through a home-made 30-interdigital finger mask (widths of 210 μm, interspaces of 70 μm). The thermal evaporation rate of Au was controlled at 2.0 Å s −1 and the chamber pressure was 3.75 × 10 −6 Torr. The patterns of MPG microelectrodes on Si wafer were then created by oxidative etching of the exposed graphene in an O 2 -plasma cleaner (Plasma System 200-G, Technics Plamsa GmbH) for 2–5 min (dependent on the thickness) with 20 sccm O 2 flow (chamber pressure 0.15 Torr) and 100–200 W rf power under the vacuum of less than 0.05 mbar. Thereafter, 5 μl H 2 SO 4 /PVA gel electrolyte was drop-casted onto the surface of interdigital electrode and solidified overnight. Finally, on-chip all solid-state MPG-MSCs with an in-plane geometry was obtained. For comparison, the TG film was prepared under the similar experimental condition (700 °C for 20 s) without using methane–plasma treatment, and the cell assembly of TG-MSCs was kept the same as that of MPG-MSCs. In parallel, all solid-state flexible MPG-MSCs were fabricated on PET substrate. A Cu foil (25 μm thick, 99.8%, Alfa Aesar) was employed as a sacrificial support and PET substrate as a flexible support. Except the transfer process, other steps were kept the same as the MPG-MSCs on silicon wafer as described above. Specifically, the transfer of graphene from Cu foil to PET substrate is as follows: first, the polymethyl methacrylate (PMMA; 950 PMMA C2, MicroChem) solution was spin-coated at 2,000 r.p.m. for 60 s on the top surface of MPG film on Cu foil (fixed on Si wafer) and annealed at 80 °C for 2 min to achieve the cure of the polymer; second, the Cu foil was etched away in aqueous Fe(NO 3 ) 3 (0.1 g ml −1 ) solution for overnight; third, the floated MPG film on PMMA support was transferred to a deionized water bath, rinsed several times by deionized water and isopropanol to fully wash off residual Cu etchant, and then the film was transferred onto the target PET substrate. Finally, the PMMA/graphene/PET film was exposed to acetone vapor at 75 °C for 1 h to remove the PMMA layer, and then rinsed with isopropanol several times. Materials characterization Materials characterization were conducted by SEM (Gemini 1530 LEO), optical microscopy, atomic force microscopy (Veeco Dimension 3100), surface profiler (KLA Tencor P-16+), X-ray diffraction (SEIFERT XRD 3000TT Bragg–Brentano diffractometer with Cu Ka radiation between 10 and 60° and an incident wavelength of 0.15418, nm), Raman spectra (Bruker, 532 nm) and X-ray photoelectron spectroscopy (Omicron Multiprobe equipped with the monochromatic Al K α source, electron analyser resolution of 0.9 eV). The electrical conductivity of the films of MPG and TG was calculated using the following equation (1): Where S is the electrical conductivity (in S cm −1 ), is the film resistance ( ) measured by a standard four-point probe system with a Kiethley 2700 Multimeter and is the film thickness (in nm). Electrochemical characterization CV examined at the scan rates of 0.01–1,000 V s −1 and EIS recorded in the frequency range of 1–100 kHz with a 5 mV ac amplitude were carried out based on a CHI 760D electrochemical workstation. The H 2 SO 4 /PVA gel electrolyte was prepared by mixing 6 g H 2 SO 4 and 6 g PVA (Mw=85,000–124,000, Sigma Aldrich) in 60 ml deionized water and heated up to 80 °C for 1 h under vigorous stirring [30] . Calculations The capacitance values were calculated from the CV data according to the following equation (2): Where is denoted as the capacitance contribution from graphene electrodes ( Supplementary Fig. S22 , Supplementary Note 2 ), is the scan rate (in V s −1 ), and are the integration potential limits of the voltammetric curve and is the voltammetric discharge current (in amperes). Specific capacitances were calculated based on the area or the volume of the device stack according to the following formula: Where (in F cm −2 ) and (in F cm −3 ) refer to the area capacitance and volumetric stack capacitance of device, respectively. A and V are the total area (cm 2 ) and volume (cm 3 ) of the device, respectively. The area capacitances were calculated based on the entire projected surface area of the device, including the area of microelectrodes and the interspaces between them. The volumetric stack capacitances were calculated by taking into account the whole volume of the device, including the volume of graphene electrodes, the interspaces between the electrodes, Au current collectors, gel electrolyte and electrolyte separators. The electrochemical performance of all solid-state devices shown in the Ragone plot was based on the volumetric stack capacitance and measured under the same dynamic condition from the discharge curves of cyclic voltammetry. The energy density of the device was obtained from the formula given in equation 5: where E is the energy density (in Wh cm −3 ), is the volumetric stack capacitance obtained from equation 3 and is the discharge voltage range (in volts). The power density of the device was calculated from the formula given in equation 6: where P is the power density (in W cm −3 ), E is the volumetric energy density obtained from equation 4 and is the discharge time (in seconds). How to cite this article: Wu, Z–S. et al . Graphene-based in-plane micro-supercapacitors with high power and energy densities. Nat. Commun. 4:2487 doi: 10.1038/ncomms3487 (2013).